Insc:LGN tetramers promote asymmetric divisions of mammary stem cells Asymmetric cell divisions balance stem cell proliferation and differentiation to sustain tissue morphogenesis and homeostasis. During asymmetric divisions, fate determinants and niche contacts segregate unequally between daughters, but little is known on how this is achieved mechanistically. In Drosophila neuroblasts and murine mammary stem cells, the association of the spindle orientation protein LGN with the stem cell adaptor Inscuteable has been connected to asymmetry. Here we report the crystal structure of Drosophila LGN in complex with the asymmetric domain of Inscuteable, which reveals a tetrameric arrangement of intertwined molecules. We show that Insc:LGN tetramers constitute stable cores of Par3–Insc-LGN-Gαi GDP complexes, which cannot be dissociated by NuMA. In mammary stem cells, the asymmetric domain of Insc bound to LGN:Gαi GDP suffices to drive asymmetric fate, and reverts aberrant symmetric divisions induced by p53 loss. We suggest a novel role for the Insc-bound pool of LGN acting independently of microtubule motors to promote asymmetric fate specification. Stem cells have the remarkable ability to self-renew, meaning that upon asymmetric divisions they generate one daughter endowed with the same stem-like property of the mother, and another one prone to differentiate. Asymmetric cell divisions (ACDs in the following) are attained by unequal segregation of cell fate defining components, and by differential positioning of siblings within the tissue. Converging evidence revealed that in several stem cell systems, only daughters retaining contact to specialized microenvironment called niches maintain stemness [1] . Mechanistically, ACDs require the coordination of the division plane, and hence the mitotic spindle axis, with polarized cortical domains. Basic mechanism of spindle coupling to cortical polarity in ACDs have been elucidated in Drosophila neuroblasts and Sensory-Organ-Precursors [2] , and found conserved in vertebrate stem cell systems including skin [3] , [4] and neural progenitors [5] , [6] , and more recently murine mammary cap cells [7] . In epithelial stem cells, apico-basal polarity is established by enrichment of the polarity proteins Par3:Par6:aPKC at the apical site, which are able to recruit at the apical membrane an adaptor named Inscuteable (Insc). Insc was first identified in larval Drosophila neuroblasts as a partner of Par3 (Bazooka in flies), and later shown to bind the switch protein Pins (the fly orthologue of LGN, referred to as dLGN in the following) [8] . Mammalian homologs of fly Insc endowed with similar properties have been discovered in mouse developing skin [3] , radial glia [9] , and mammary stem cells [7] , and are required for the correct execution of oriented ACDs. LGN in turns binds directly to the Dynein-associated protein NuMA with its tetratrico-peptide repeat (TPR) domain (hereon LGN TPR ) and to multiple Gαi subunits of heterotrimeric G-proteins, whose myristoyl group inserts into the lipid bilayer. During ACDs, the minus-end directed movement of Dynein engaged at the apical membrane with NuMA and LGN results in pulling forces on astral microtubules able to align the mitotic spindle along to the apico-basal polarity axis. Based on its interaction with both Par3 and LGN, and its involvement in oriented ACDs, Insc has long been considered the molecular connection between the polarity proteins Par3:Par6:aPKC and the spindle tethering machinery assembled on Dynein-NuMA:LGN:Gαi. Recent evidence indicate that Insc and NuMA are mutually exclusive interactors of LGN [10] , [11] raising the question as to how molecularly Insc works in ACDs. The mammary gland is a branched ductal system consisting of a luminal epithelial layer surrounded by a myoepithelial contractile layer, embedded in a stromal matrix. In mammals, mammary gland development peaks at puberty and is driven by terminal end bud structures (TEBs) that forms at tips of the growing ducts and proliferate rapidly into the fat pad. TEBs in turn are composed by an outer basal layer, and multiple inner layers of luminal epithelial body cells. The regeneration cycles observed in mammary glands at pregnancies are sustained by mammary stem cells (MaSCs) residing in the TEBs [12] , which have been shown to self-renew in an Insc-dependent manner [7] , [13] . More specifically, in mice during puberty, cap cells undergo mitosis with NuMA and LGN crescents polarized above one of the spindle poles [7] , [14] . Interestingly, although the existence of multipotent mammary stem cells in adult mice seems unlikely [15] , it has been shown that mammary epithelial cells isolated from murine mammary gland gain stemness in vitro and exhibit pluripotency. Insc has been reported to promote ACDs also in Drosophila neuroblasts, murine skin progenitors and neural stem cells [6] , [16] , [17] , [18] . Structural studies revealed that Insc codes for a conserved 35-residue peptide (Insc PEPT hereon) binding to the N-terminal TPR domain of LGN/dLGN with nanomolar affinity [10] , [11] , [19] . Beside Insc PEPT , vertebrate and invertebrate orthologues of Insc share poor sequence homology. Both proteins are predicted to contain a helical rich region downstream of the LGN-binding peptide, which in the case of the Drosophila Insc is sufficient to recapitulate its localization and functions in asymmetric divisions of neuroblast (hence termed Insc ASYM ) [20] , [21] . No structure-function analysis is to date available for human Insc besides N-terminal truncations shown to impair binding to LGN [9] . Intriguingly, in vitro human Insc has been reported to interact with the PDZ domains of Par3 via a conserved C-terminal motif [22] , [23] , outside of the central helical fragment. To understand the molecular basis of Insc functioning, we set out to study the organizational principles of the Par3–Insc–LGN–Gαi interaction, and their impact on murine mammary stem cell asymmetric divisions. Our studies revealed that LGN and Insc form stable tetramers at the core of Par3–Insc–LGN–Gαi macromolecular assemblies, which are required for asymmetric fate acquisition of MaSCs, and do not exchange LGN molecules with microtubule motors. Molecular architecture of the dLGN TPR :Insc ASYM tetramer Previous structural studies have revealed that the flexible Insc PEPT binds to the inner side of the TPR α-solenoid of LGN/dLGN with an extended conformation [10] , [19] . To determine the atomic model of the whole Insc ASYM , we took advantage of a discistronic pGEX vector co-expressing GST-dLGN 25–406 with the Drosophila Insc ASYM construct encompassing residues 283–623 (Supplementary Fig. 1a ). The structure of dLGN TPR :Insc ASYM was solved by molecular replacement using the coordinates of dLGN TPR :Insc PEPT as a search model. Multi-crystal averaging was employed to obtain an interpretable electron density for manual model building of the Insc ASYM domain. 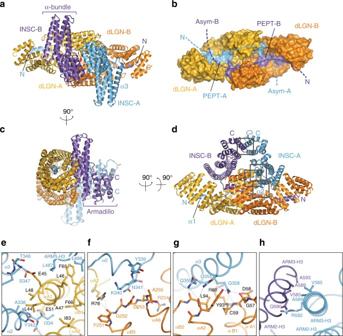Fig. 1 Structure of the dLGNTPR:InscASYMcomplex.a–dCartoon representation of the dLGNTPR:InscASYMtetramer in three orthogonal orientations. The two protomers of dLGNTPRare colored gold and orange, while the two InscASYMare in cyan and purple. The two-fold symmetry axis of the tetramer is marked as a red oval ina.bSurface representation of the arrangement of the dLGNTPRdomains with the N-terminal fragments of InscASYM-labeled PEPT (InscPEPTin the text) in the same orientation and colors as ina.e–hClose-up views of the interaction of Insc-Awith the other subunits of the tetramer from the N terminus to the end of the polypeptide chain. The positions of the individual close-up views within the complex are indicated ind. Interacting residues at the interfaces are depicted in balls-and-sticks The final model was refined at 3.4 Å resolution to an R free of 25.0% and R work of 20.9% with good stereochemistry (Table 1 and Supplementary Fig. 1b, c ). It consists of residues 41–386 of dLGN and residues 302–595 of Insc ASYM , thus lacking about 20 residues preceding the Insc PEPT stretch. Table 1 Data collection and refinement statistics Full size table The most striking feature of the dLGN TPR :Insc ASYM structure lies in its hetero-tetrameric arrangement (Fig. 1a ), whereby each Insc chain contacts one dLGN TPR with the elongated Insc PEPT stretch and the second dLGN TPR with a four-helix bundle, in a sort of intimate domain-swap (Fig. 1b ). The C-terminal portion of the Insc ASYM chains protrudes away from the TPR domains, and folds in Armadillo units, packing to one another via the last helices of the repeat (Fig. 1c, d ). In the tetramer, the two dLGN TPR molecules form homotypic head-to-head interactions by shape complementarity mediated by the linkers joining TPR3-4-5 of the two subunits. Topologically, this packing of the TPR domains does not prolong the super-helical array of consecutive TPR motifs, but rather generate a cylindrical scaffold entirely closed on one side (Fig. 1b ). The two Insc PEPT fragments run antiparallel to one another lining along the inner side the TPR channel, whose open side is occupied by the helical bundles of the Insc ASYM folds (Fig. 1c ). This way, each Insc ASYM chain precludes solvent accessibility to the dLGN TPR molecule to which it is not in contact with its own Insc PEPT . The extended tetramer interface generated by a non-crystallographic two-fold axis roughly passing through the helical domains of Insc ASYM buries a surface of about 8000 A 2 (Fig. 1a ). Interestingly, self-association of TPR domains has been reported for several components of the Anaphase-Promoting Complex (APC), the E3-ligase driving mitotic exit [24] . However, APC subunits homodimerize by hooking of the N-terminal TPRs, which engage in a tight clasp-like interaction [25] , whereas dLGN TPR protomers are monomeric in isolation and dimerize only in the presence of Insc ligands longer than the peptide fragment (Supplementary Fig. 2 ). Fig. 1 Structure of the dLGN TPR :Insc ASYM complex. a–d Cartoon representation of the dLGN TPR :Insc ASYM tetramer in three orthogonal orientations. The two protomers of dLGN TPR are colored gold and orange, while the two Insc ASYM are in cyan and purple. The two-fold symmetry axis of the tetramer is marked as a red oval in a . b Surface representation of the arrangement of the dLGN TPR domains with the N-terminal fragments of Insc ASYM -labeled PEPT (Insc PEPT in the text) in the same orientation and colors as in a . e–h Close-up views of the interaction of Insc- A with the other subunits of the tetramer from the N terminus to the end of the polypeptide chain. The positions of the individual close-up views within the complex are indicated in d . Interacting residues at the interfaces are depicted in balls-and-sticks Full size image Looking from the side of the TPR domains, the dLGN:Insc tetramer resembles a sailing boat (Fig. 1d ), whose hull is formed by the TPR scaffolds and sails by the helical domains of Insc ASYM . The symmetrical arrangement of the tetramer is reflected in equivalent interactions among the subunits. To facilitate the description we will name the dLGN and Insc couples interacting via the Insc PEPT as A and B . Several conserved hydrophobic and polar interactions between Insc PEPT and dLGN TPR account for the nanomolar binding affinity of the binary interaction [10] , [11] , [19] . The Insc PEPT stretch of Insc- A ASYM lines along the inner dLGN- A TPR surface as seen in the dLGN TPR :Insc PEPT structure. Remarkably, in the tetramer, residues 334–342 of Insc- A PEPT fold into a second α2-helix that packs parallel to the αA1–αA2 helixes of dLGN- A TPR with primarily hydrophobic interactions (Fig. 1e and Supplementary Movie 1 ). This α2-helix of Insc- A ASYM is capped by TPR5-6 of dLGN- B TPR , in an interaction contributed by hydrogen bonds between Lys340-Asn341 Insc-A and Gly252-Asp253-Ala255 dLGN-B (Fig. 1f ). After wedging between the two TPR domains, the Insc- A ASYM chain undergoes an abrupt kink to form the first helix of the bundle (the α3 helix of Insc ASYM , Fig. 1a ), running almost orthogonal to the dLGN- A TPR repeats. Compared to the extensive contacts engaging the Insc PEPT , fewer specific interactions are found in the rest of the interface between Insc and dLGN molecules. A cluster of Gln residues in the middle of the α3 helix of Insc- A ASYM packs against the intra-repeat loops of the TPR1-2 dLGN-B making bidentate hydrogen bonds with main chain atoms and staking interactions with Tyr93 dLGN-B (Fig. 1g ). These contacts create a topological closure of the TPR channel. In the center of the tetramer hull, the symmetrical interface between dLGN- A TPR and dLGN- B TPR is contributed primarily by hydrogen bonds between main chain atoms of TPR turns, as exemplified at TPR4-5 (Supplementary Fig. 3a, b ). The corresponding interface at the tip of the sails is maintained by pairing of the α3-helices of the third Armadillo repeats via hydrophobic interactions between Val585 Insc and Ala589 Insc of both chains, further strengthened by a polar interaction between Arg582 Insc-A and Gln590 Insc-B (Fig. 1h and Supplementary Movie 1). Thus, based on structural evidence, we can conclude that (1) the dLGN TPR :Insc ASYM is a symmetrical tetramer of intertwined subunits, whose high affinity binding is dictated by extended interactions between the Insc PEPT and the TPR domains; (2) the helical portions of the Insc ASYM chains introduce into the tetramers a topological constrain preventing the dissociation of the complex. Conformational flexibility of the Pins:Insc tetramers Insc works in complexes localized in proximity of the plasma membrane, which is an inherently flexible structure. Consistent with this role, we found that the four independent copies of the tetramer present in the asymmetric unit display two slightly different conformations, one extended (described in the previous paragraph) and the other more compact. Comparison of the two classes of tetramers revealed the existence of a structurally invariant rigid body including one of the dLGN TPR domains (referred to as dLGN- A TPR in the following), and the cognate Insc- A PEPT . Upon superposition on this rigid body, a major rearrangement at the C-terminal end of dLGN- B TPR becomes visible (Fig. 2a ). The compaction of the tetramer hull is transmitted allosterically to the Insc- A ASYM domain, whose helical bundle is disrupted to accommodate TPR7-8 of dLGN- B (Fig. 2b–d , Supplementary 3a–d and Supplementary Movie 2 ). To assess whether the structural variability observed in the crystal packing is preserved in solution, we performed SEC-SAXS analyses of the complex. The low-resolution ab initio shape determined from the experimental data provided a particle envelope consistent with the tetramer (Fig. 2e–f and Supplementary Fig. 3f ), with a radius of gyration R g of about 41 Å, and maximum particle size D max of 120 Å. Interestingly, the experimental data deviates substantially from the scattering pattern calculated from extended and compact tetramers individually (discrepancy χ 2 in the order of 8.0), suggesting that in solution these assemblies are flexible and free to sample a conformational space including, but not limited, to the arrangements observed in the crystals. We conclude that the dLGN TPR :Insc ASYM tetramer is endowed with an intrinsic structural plasticity mirroring the extended and compact organization of the crystallographic structures. Fig. 2 The dLGN TPR :Insc ASYM complex adopts two conformations. a Superposition of the two dLGN TPR :Insc ASYM conformers present in the a.s.u. The most compact conformer is shown as ribbon diagram, and the most extended is depicted in transparent cylindrical helices. Subunits are colored as in Fig. 1 . b , c Zoomed views of the interfaces between the helical bundle of Insc- A and TPR7-8 of dLGN- B for the compact (top) and extended (bottom) tetramers. The rearrangement of the TPR repeats of dLGN-B in the compact conformation is accompanied by disruption of the initial turns of helix α5 of Insc- A . d Graphical summary of the conformational changes between the extended and the compact tetramers. e SAXS data for the dLGN TPR :Insc ASYM complex in comparison to the theoretical curves for the different configurations (upper part and inlay) and fits of ab initio models in P1 (gray) and P2 symmetry (blue). Idealized curves were obtained merging frames with matching radius of gyration and high similarity according to CORMAP [38] , [39] . f The ab initio model of the dLGN TPR :Insc ASYM complex in P1 symmetry (transparent gray spheres) matches well with both the extended (orange) and compact (green) tetramers Full size image Conserved topology of the Insc ASYM domain A great challenge in the stem cell field deals with the understanding of the molecular mechanism accounting for vertebrate asymmetric cell divisions. Human Insc was identified as a protein endowed with the same interaction properties and spindle orientation functions of fly Insc. Nonetheless invertebrate and vertebrate Insc orthologues share very poor sequence homology (Fig. 3g and Supplementary Fig. 4 ). To understand whether the architecture of the dLGN TPR :Insc ASYM oligomers recapitulate the organizational principles of human counterparts, we carried out a comparative analysis of Insc in the two species, starting from the topology of the asymmetric domain. After the TPR-interacting peptide, Drosophila Insc ASYM forms an elongated helical bundle, followed by a globular domain of three Armadillo (ARM) repeats (Fig. 3a, b ). Each ARM unit consists of two short helices followed by a long one, designated H1, H2, and H3. In fly Insc ASYM , the first ARM is contributed by the C-terminal half of helix-α6, which bends to conform to the orientation of ARM helices H1 and H2 (Fig. 3b ). Insertion of Phe506 Insc into a hydrophobic pocket organized by Leu and Phe residues of helices α-4 and α-6 of the bundle maintains the ARM domain orthogonal to the helical bundle (Fig. 3c ). To define whether human Insc adopt the same structure, we compared its secondary structure prediction with the experimentally defined helical pattern of Drosophila Insc ASYM , and found that the fragment of about 300 residues after the human Insc PEPT is predicted to assume a helical conformation with a sequence of short and long elements consistent with the fly Insc ASYM fold (Fig. 3g ), suggesting that the two Insc orthologues fold similarly. We then asked whether human Insc could oligomerize with LGN TPR . To this end, we purified to homogeneity the human LGN TPR :Insc complex expressed recombinantly in insect cells from a dicistronic baculovirus vector. In line with the crystallographic and SAXS data, Static-Light-Scattering analysis confirmed that the Drosophila dLGN TPR :Insc ASYM complex elutes from a size-exclusion column as a tetramer (Fig. 3d ). When loaded on a size-exclusion column, the human LGN TPR :Insc complex elutes slightly earlier than the dLGN TPR :Insc ASYM tetramer (Fig. 3e ), and before the 158 kDa molecular weight marker, indicating that its most abundant oligomeric state is a 2:2 hetero-tetramer. We reasoned that the difference in the elution profiles of fly and human assemblies could be ascribed to the longer human Insc full-length construct (about 58 kDa in size) as compared to the Drosophila Insc ASYM (about 33 kDa). To further corroborate the idea that human LGN and Insc form hetero-tetramers, we co-transfected HEK293T cells with two differentially tagged versions of LGN TPR (Flag-LGN TPR and GFP-LGN TPR ) together with Insc ASYM or a variant of Insc ASYM lacking the region spanning residues 62–191 that corresponds to the four-helix bundle (hereon referred to as Insc ASYM -ΔαB). To improve detection in immunoblot, in this experiment we used GFP-tagged Insc ASYM -ΔαB. Flag-tagged human LGN TPR co-immunoprecipitates GFP- LGN TPR in the presence of Insc ASYM , whereas in the presence of Insc ASYM -ΔαB it does not (Fig. 3f ). Consistently, the LGN TPR :Insc ASYM complex elutes earlier from a SEC column than the LGN TPR :Insc ASYM -ΔαB complex (Supplementary Fig. 3g ), confirming that Insc ASYM -ΔαB assemble in a lower stoichiometry complex than wild-type Insc. We conclude that (1) fly and human Insc ASYM are likely to share the same helical topology; (2) human Insc tetramerizes with LGN TPR ; and (3) removal of the α-bundle results in the destablilization of the tetrameric assembly with a human Insc ASYM mutant associating with LGN TPR in a 1:1 stoichiometry. Fig. 3 The topology of the asymmetric domain of Insc is evolutionary conserved. a , b Cartoon model of Insc ASYM bound to the inner groove of dLGN TPR (in white) at two orthogonal views. After the initial Insc PEPT stretch (in cyan), the Insc chain departs from the TPR α-solenoid forming a four-helix bundle (green). The C-terminal part of the last helix of the bundle kinks into two short helical fragments of the first non-canonical ARM repeat (gold), which is followed by two conventional ARM motifs adopting a triangular flat shape (pink and brown). c Zoom of the hydrophobic pocket in which Phe506 Insc fits. d Static-Light-Scattering profile of the dLGN TPR :Insc ASYM tetramer showing an average molecular mass of about 180 kDa along the peak, as expected for a 2:2 tetramer. e SEC elution profiles of Drosophila dLGN TPR :Insc ASYM (blue trace) and human LGN TPR :Insc (green trace) with associated Coomassie-stained SDS–PAGE separation of peak fractions. The elution profile of globular markers is reported in a dashed gray line. Both complexes elute in fractions consistent with the theoretical molecular mass of 2:2 tetramers. f Insc ASYM -ΔαB assembles with LGN TPR in a 1:1 stoichiometry. HEK293T cells were transiently transfected with plasmids containing human GFP-LGN TPR and FLAG-LGN TPR (residues 1–350) alone or in combination with human Insc ASYM or Insc ASYM -ΔαB (lacking residues 62–191). After 48 h, cells lysates were immunoprecipitated (IPs) with anti-FLAG antibodies conjugated to sepharose beads, and immunoblotted (IB) with the indicated antibodies. FLAG-LGN TPR - was able to co-immunoprecipitate with GFP-LGN TPR only when bound to Insc ASYM , but not to Insc ASYM -ΔαB. g Sequence alignment of Insc ASYM with secondary structure elements based on the crystallographic structure (for Drosophila ) and in silico prediction (for Homo sapiens ). Residues are colored according to the degree of conservation calculated on the basis of the alignment of Supplementary Fig. 4 . Circles indicate residues of Insc ASYM in contact with the other three subunits of the tetramer Full size image Organizational principles of the Par3:Insc:LGN:Gαi complexes Establishing apico-basal polarity is a prerequisite for asymmetric cell divisions. An evolutionary conserved function of Par3 has been described in marking the apical site of polarized mitoses, and conferring fate specification upon inheritance. In most instances Insc and LGN are found polarized with Par3 [16] , [26] , [27] . In embryonic epidermis endogenous Insc and Par3 co-immunoprecipitate [3] . Similarly, human Insc and Par3 co-transfected in HEK293T cells co-immunoprecipitate via a direct interaction between the C terminus of Insc and the PDZ domains of Par3 [23] (Supplementary Fig. 5a–c ). Interestingly the whole PDZ domain of Par3 is required for binding to Insc (Supplementary Fig. 5d ). The identification of distinct regions of Insc binding to Par3 and LGN prompted us to ask whether Insc is the direct physical link between LGN and the polarity complex. Immunoprecipitation of LGN from mitotic lysates co-expressing Par3 in the presence or in the absence of Insc revealed that Insc is required for the association of LGN with Par3 (Fig. 4a ). Consistently, the recombinant Par3 PDZ123 domain binds to the Insc:LGN:Gαi assembly purified from insect cells with a stoichiometry reflecting the amount of Insc, and elutes for a SEC column right after the 670 kDa marker, in agreement with the theoretical molecular weight of an oligomer containing two copies of Insc and LGN (Fig. 4b ). Collectively these findings demonstrate that the apical complex Par3:Insc:LGN:Gαi is held together by direct interactions centered on Insc:LGN tetramers, and connected to the plasma by Par3 and Gαi (Fig. 4c ). Fig. 4 Conserved organizational principles of Par3:Insc:LGN:Gαi complexes. a Reconstitution of human Par3:Insc:LGN interaction in cells. HEK293T cells were transfected with Par3-GFP, FLAG-LGN and HA-Insc. Cell lysates were subjected to IP with α-FLAG antibody conjugated to sepharose beads. After washes, species on beads were analyzed by SDS–PAGE and immunoblotted as indicated in the figure. HA-empty vector was included as a negative control of the IP. b SEC elution profiles and SDS–PAGE separation of Insc:LGN:Gαi complexes reconstituted from expression in insect cells (dark green trace) and Par3 PDZ123 purified from bacterial sources (pink trace). When the Par3 PDZ123 is mixed in molar excess with Insc:LGN:Gαi, it coelutes with Insc:LGN:Gαi in a stoichiometry reflecting the amount of Insc in the complex (light green trace). c Summary of the interactions in the Par3:Insc:LGN:Gαi complex supported by our study. Stable Insc:LGN tetramers form the core of apically localized Par3:Insc:LGN:Gαi complexes, in which the C-terminal portion of the two Insc chains contacts directly the PDZ domains of Par3. Binding of each LGN-GoLoco to four Gαi GDP molecules stabilizes the association of the macromolecular assemblies to the plasma membrane Full size image Relevance of the Insc:LGN topology for breast stem cell ACD To assess the functional relevance of the Insc:LGN tetramers, we investigated the in vitro self-renewal of murine mammary stem cells (MaSCs) ectopically expressing Insc fragments designed on the basis of the structural analyses. Although cultured mammary epithelial cells may not fully reflect the properties of mammary stem cells residing in the mammary glands [15] , we reasoned that in vitro analyses of isolated murine MaSCs could be used to dissect molecular mechanisms of cell division decoupled from niche signals. More specifically, previous studies reported that the first division of MaSCs isolated from wild-type mice is most frequently asymmetric, whereas the division mode of MaSCs derived from p53-KO mice is for the large majority symmetrical, eventually leading to the expansion of the SC compartment [28] . MaSCs from primary tissues of human and mouse origin can be grown in vitro in non-adherent conditions, giving rise to clonal spheroids called mammospheres [29] . In these assays, the number of mammospheres reflects the number of MaSCs originally present in the culture. MaSCs from the p53-KO mice expands aberrantly in culture as consequence of their symmetric mode of division, increasing the number of mammospheres observed over serial propagation [28] , [30] . Interestingly, qPCR analysis revealed that the Insc transcript is absent in p53-KO mammospheres (Fig. 5a ), whereas Par3, LGN and NuMA are still transcribed (Supplementary Fig. 6a–c ). Thus we reasoned that p53-KO MaSCs would be the ideal experimental setting to test whether Insc promotes asymmetry by reverting the symmetric division mode induced by p53 loss. We then infected p53-KO mammospheres with a lentiviral vector restoring the amount of full-length human Insc transcript at levels comparable to the endogenous one in wild-type MaSCs (Fig. 5a ), and analyzed the division mode of MaSCs. Immunofluorescence analysis of doublets with the basal cell surface marker CD49f (ITGA6) showed that Insc-expressing MaSCs partition CD49f unequally (Fig. 5b, c ), consistent with the role of Insc as determinant of ACD documented in other vertebrate stem cell systems [6] , [16] , [17] . Most importantly, in cultured MaSCs CD49f and Numb co-partition asymmetrically (Supplementary Fig. 6d ), further corroborating the notion that in this system, ectopic expression of Insc promotes asymmetry. The increased proportion of ACDs versus SCDs observed in Insc-expressing p53-KO MaSCs predicts a reduction in their self-renewal capacity (Fig. 5d ). To test this hypothesis, we set out to perform a serial propagation experiment using mammospheres from p53-KO mice infected with full-length Insc. Indeed, the sphere-forming efficiency (SFE) of p53-KO mammospheres infected with Insc displayed a 70% decrease, indicating a reduced clonogenic ability of the Insc-expressing MaSCs upon three serial passages (Fig. 5e ). Notably, Insc ectopic over-expression does not perturb LGN, NuMA and Par3 levels (Supplementary Fig. 6a–c ), indicating that the Par3:Insc:LGN complex and the spindle orientation motors works physiologically. To dissect the molecular requirements for the reduced self-renewal induced by Insc, we repeated the mammosphere assays expressing human Insc ASYM , spanning residues 1–317, which tetramerizes but is unable to bind Par3, or Insc PEPT , sufficient for binding to LGN but not for oligomerization. SFE analyses revealed that comparable expression of Insc ASYM decreases self-renewal of p53-KO MaSCs to the same extent of full-length Insc, whereas Insc PEPT does not (Fig. 5f–h and Supplementary 6e, f ). Mammospheres grown from MaSCs infected with different Insc constructs displayed the same surface area and GFP-reporter intensity, which remained unchanged upon the three analyzed passages, thus excluding proliferative defects or toxicity induced by lentiviral transduction (Fig. 5g, h ). Importantly, inability to revert SCDs of p53-KO MaSCs in SFE assays was also observed upon lentiviral expression of the Insc ASYM -ΔαB mutant forming 1:1 complexes with LGN (Fig. 5i and Supplementary 6g ), further corroborating the notion that binding of Insc to LGN is not sufficient to promote ACDs, and that the terameric arrangement is key to mediate asymmetry. Fig. 5 Insc ASYM induces ACDs in p53-KO mammary stem cells. a Insc transcript levels evaluated by RT–qPCR on mammospheres from wild-type FVB mice, or p53-KO mice infected with empty lentivirus (EV) or human full-length Insc (INSC) normalized to the Rpp0 control. Bars represent mean ± s.d. of three replicates. Statistics for 1 out of 2 independent experiments. b , c Images and quantification of the division mode of mammary epithelial cells from p53-KO mice evaluated by pair-cell assay. Cell infected with empty lentivirus (EV) or virus expressing full-length Insc (INSC) were stained with CD49f and DAPI. Scale bar, 10 μm. Quantification from 2 independent experiments with n > 10 cells for all conditions in each experiment. p = 0.005 according to the paired Student’s test. d Scheme of the SFE assay used to evaluate self-renewal of p53-KO MaSCs. Stem cells are in blue, progenitors in pink. e Number of mammospheres from p53-KO mice infected with an empty lentivirus (EV) or a virus expressing Insc (INSC) counted over three serial passages and shown by box-plots with mean of 10 wells count per each passage (green line). f – h SFE assays with p53-KO mammospheres infected with empty virus (EV) or viruses expressing Insc (FL), Insc ASYM (aa 1–317, ASYM), or Insc PEPT (aa 1–58, PEPT). For each passage, the number of spheres ( f ), the sphere area ( g ) and the GFP intensity ( h ) have been evaluated for 10 wells, and plotted as in e (each pair Student’s t -test). Statistics for 1 out of 3 independent experiments. i SFE assays performed with p53-KO mammospheres infected with empty lentivirus (EV) or viruses expressing Insc (FL), Insc ASYM (ASYM), or Insc ASYM -ΔαB (i.e. Insc ASYM lacking aa 62–191). For each passage, the number of spheres has been counted for four wells, and plotted as above (each pair Student’s t-test). Statistics for one out of two independent experiments. j SFE assays performed with p53-KO mammospheres infected with empty lentivirus (EV) or viruses expressing Insc (FL), human LGN-GoLoco (aa 358–677) or both. For each passage, the number of spheres has been evaluated in three wells, and plotted as above (each pair Student’s t -test). In the figure, * P < 0.01, *** P < 0.001 by Wilcoxon’s test Full size image In most of ACDs characterized so far, Insc polarizes with LGN at the apical site by direct interaction with the membrane-associated proteins Gαi and Par3 [16] , according to the topology that we characterized in the previous paragraph. To understand the relevance of Gαi in Insc-mediated ACDs, we conducted a SFE assay co-infecting p53-KO MaSCs with full-length Insc and a dominant-negative variant of LGN coding only for the C-terminal GoLoco region, which retains binding to Gαi but not to Insc, this way titrating away Insc:LGN complexes from the plasma membrane. In the presence of the LGN-GoLoco, Insc fails to reduce the sphere number in SFE assays (Fig. 5l and Supplementary Fig. 6h, i ), demonstrating that the Gαi tethering of tetramers to the plasma membrane is a prerequisite for ACDs. Collectively, these data showed that restoring Insc levels in p53-KO MaSCs reverts symmetric divisions towards asymmetric ones and restricts self-renewal, and that the Insc ASYM -mediated tetramerization of Insc with Gαi-bound LGN is essential for these functions. The finding that Insc engages LGN in a stable tetramer, and that this interaction is competitive with the binding of LGN to the Dynein-adaptor NuMA [10] , [11] , poses the question of how the Insc-bound and NuMA-bound pools of LGN relate to one another during ACDs. To gain a first insight into the relative abundance of LGN and Insc, we analyzed their transcript levels in human mammary epithelial CD44 high /CD24 low cells isolated from HMLE cell line (immortalized human mammary epithelial cells), which exhibit properties of MaSCs [31] . Human mammary CD44 high /CD24 low cells express significantly higher levels of Insc compared to the CD44 low /CD24 high non-stem counterpart (about 2.5-fold) and LGN expression was far more abundant than Insc (Supplementary Fig. 6l ). Although we cannot exclude that Insc and LGN protein levels are post-transcriptionally regulated, these data seem to suggest that Insc acts as limiting factor in the Insc:LGN complex formation. Because Insc forms stable tetramers with LGN, we can assume that NuMA is unable to prevent the formation and the activity of Insc:LGN tetramers in spite of competing with Insc for LGN binding and being more abundant. Conversely, since Insc is much less expressed than LGN, Insc:LGN complexes do not alter the spindle orientation functions exerted by LGN in complex with NuMA/Dynein, but rather play a specific role that is essential for asymmetric stem cell divisions. The current view posits that LGN contributes to asymmetric fate of oriented stem cell divisions by recruiting microtubule motors at the apical site via direct interaction with NuMA. Although LGN is clearly important to coordinate cortical polarity with mitotic spindle orientation, in this paper we show that a pool of LGN is engaged in a stable oligomeric assembly with Insc, Par3, and Gαi, which cannot exchange with NuMA. We speculate that this complex underpins a novel and conserved function of cortical Par3:Insc:LGN:Gαi complexes in promoting asymmetry by stabilizing fate defining components at the apical site, which is partitioned unequally upon cytokinesis. Insc was originally identified in fly neuroblasts as an adaptor binding to dLGN. Previous structural studies showed that the short Insc PEPT (residues 304–340) binds to the dLGN TPR domain with nanomolar affinity, leaving open the issue as to why only a larger Insc fragment (termed Insc ASYM ) was required to recapitulate its functions in Insc-deficient neuroblasts [21] , [32] . The crystallographic structure of the dLGN TPR :Insc ASYM complex reveals that Insc ASYM induces a stable dimerization of the dLGN TPR domains, which topologically prevents the dissociation of the two molecules. Together, these findings imply that the asymmetric function of the dLGN:Insc assembly is embedded in its oligomeric form. In flies, the Insc ASYM domain develops C-terminally of the Insc PEPT in two helical domains, which have been previously assigned to specific Insc functions in neuroblasts. In particular, the fragment 302–459 roughly matching the helical bundle was shown to target Insc at the apical membrane [21] , possibly because it is sufficient to trigger tetramerization with dLGN, while the Armadillo region encompassing residues 460–552 / 578 is required to drive asymmetric distributions of Numb and Miranda [21] , [32] , for molecular reasons that still remain unclear. Based on in vitro reconstitution experiments, we cannot exclude that the Armadillo repeats contribute to the larger interface accounting for the interaction of dLGN TPR :Insc ASYM with Par3 PDZ and hence with the polarity complex (see below). An important finding of our structural studies is that the functional homology between vertebrate and invertebrate Insc is rooted in the same overall organization of the assemblies that they form with their cognate TPR-GoLoco proteins. We found that the region of human Insc spanning residues 1–316 is predicted to fold as a helical domain resembling the fly Insc ASYM , and that it forms analogous tetramers with human LGN TPR . The evidence that in fly neuroblasts mouse LGN can rescue spindle defects induced by dLGN depletion corroborates the notion that their TPR domains assemble with Insc similarly [33] . Reconstitution of the whole human Par3:Insc:LGN:Gαi complex from recombinant sources showed that Insc links physically LGN to Par3 by direct binding to its PDZ domains. As expected for canonical PDZ ligands, the conserved C-terminal tail of Insc is the prominent determinant for the binding of Insc to Par3 PDZ123 . What is the relationship between the Insc-bound pool of LGN and the spindle orientation? The topology of the stable Insc:LGN tetramer implies that the LGN molecules engaged with Insc cannot be sequentially transferred to NuMA to pull on astral microtubules, as we had previously proposed [10] , [34] . Nonetheless, we show that Insc promotes asymmetric divisions in cultured p53-KO MaSCs, consistent with previous reports in skin progenitors and radial glial cells [4] , [6] , [16] , [17] . We speculate that only a minor fraction of LGN molecules associates with Insc during ACDs, leaving the bulk of the LGN population available for the assembly of NuMA/Dynein motor complexes. In this view, the two LGN-containing complexes would contribute to asymmetry in different ways: the Insc-bound pool by coordinating the distribution of fate determinants, including Par3, and the more abundant NuMA-bound pool by providing cortical information to orient the division plane (Fig. 6a ). The evidence that fly Insc ASYM is involved in basal localization of Miranda and Pon/Numb speaks in favor of this hypothesis. Fig. 6 Model of the role of Insc:LGN complex in asymmetric divisions. a Schematic diagram depicting the organization of cortical domains and mitotic spindle motors in murine mitotic mammary stem cells. b Schematic representation of the asymmetric function of Insc:LGN tetramers supported by our study. Initally, Insc:LGN complexes are recruited at the apical membrane by direct binding of LGN to Gαi-GDP molecules, and by association of Insc with Par3. Cooperative binding to LGN-GoLoco motifs favors Gαi-GDP apical clustering. Later, a Gαi GTP-cycle, likely catalyzed by a GEF such as Ric-8A, dissociates Gαi from Insc:LGN, generating a localized pool of Gαi-GTP molecules, which upon GTP hydrolysis recruits LGN:NuMA:Dynein complexes at the apical site. According to this model, stable Insc:LGN assemblies couple asymmetric fate specification with apico-basal spindle orientation by Gαi-GDP transfer Full size image Intriguingly, mammosphere assays revealed that the Par3-binding domain of Insc, residing outside the Insc ASYM , is dispensible for ACDs, in agreement with previous findings in fly neuroblasts [21] , [32] . Conversely, binding of LGN to Gαi is essential to promote Insc-dependent MaSCs ACDs, suggesting that during ACDs Gαi likely acts as recruitment factor for Insc:LGN complexes at the apical membrane. We speculate that the Gαi GDP moieties, possibly generated by specific GPCR activities [35] , anchor Par3:Insc:LGN:Gαi complexes at a localized cortical site by direct binding to the LGN-GoLoco motifs. Because also NuMA:LGN assemblies contain Gαi GDP , we think that GDP-loaded Gαi might be the common positional cue coupling asymmetric and orientation activities of LGN during ACDs, including the ones of cultured MaSCs, keratynocites and fly neuroblasts. In spite of competing with NuMA for LGN binding, during ACDs Insc is required for correct spindle orientation [6] , [9] , [16] , [18] , [26] , [36] . To explain this phenotype, we propose that stable Insc:LGN complexes are targeted at a restricted cortical site by direct interaction with Gαi GDP , and favor clustering of Gαi by cooperative binding of each LGN-Goloco domain to four Gαi molecules. LGN associates only with the GDP-loaded form Gαi, thus it is plausible that specialized GEFs/GAPs catalyze a Gαi GTP-cycle that releases Gαi from Insc:LGN complexes and allow engagement of the same apically enriched Gαi molecules to LGN:NuMA, this way contributing to apico-basal spindle orientation (Fig. 6b ). According to this model, aberrant boosting of Insc levels in wild-type stem cells would eventually titrate away LGN from NuMA promoting misoriented symmetric divisions, as it was recently observed in MaSCs isolated from Insc knock-in mice [7] . The finding that ectopic over-expression of Insc in the developing skin results in a transient ACDs increase without morphogenetic long-term defects, indicate that feedback mechanisms exists to control the balance between ACDs and SCDs in tissues [17] . Further investigations will be needed to address the physiological relevance of our molecular findings for self-renewal of MaSCs residing in the mammary glands. Finally, a very interesting observation stemming from our mechanistical studies is that Insc replenishment in p53-KO MaSCs reverts the symmetric division phenotype induced by p53 loss. Although the molecular basis underlying such remarkable effect are currently unclear, this finding indicates that Insc acts downstream of p53 in controlling MaSCs self-renewal. As the most aggressive breast tumors arise from deregulation of MaSCs homeostasis and self-renewal [37] , and p53 is found mutated in nearly 40% of human breast cancers [28] , we anticipate that experiments addressing the mechanisms underpinning the working principles of Insc in p53-KO MaSCs in vivo might be instrumental to the development of novel therapeutical strategies targeting breast cancer stem cells. Protein preparation To generate a crystallization quality sample, the dLGN 25–444 :Insc 252–623 complex previously purified [10] was subjected to limited proteolysis, which resulted in two trimmed domains assigned by Mass Spectrometry to residues 25–406 of dLGN and residues 283–623 of Drosophila Insc. These two fragments were cloned into a dicistronic-modified version of the pGEX-6P1 vector (GE Healthcare), and co-expressed in BL21 Rosetta E . coli cells by induction with 0.5 mM IPTG overnight at 18 °C. Cells were lysed in 0.1 M Tris-HCl pH 8, 0.3 M NaCl, 10% glycerol, 0.5 mM EDTA, and 5 mM DTT, and cleared for 1 h at 100,000 g . Cleared lysates were affinity purified by incubation with Glutathione Sepharose-4 Fast-Flow beads (GE Healthcare). After washes, fusion proteins retained on beads were incubated with PreScission protease (GE Healthcare) overnight at 4 °C to remove the GST-tag. The cleaved material was eluted from the beads in a desalting buffer consisting of 20 mM Tris-HCl pH 8, 40 mM NaCl, 5% glycerol, 5 mM DTT, and loaded on Resource-Q ion-exchange columns. Peak fractions were pooled, and loaded on a Superdex-200 column equilibrated in 10 mM HEPES pH 7.5, 0.6 M NaCl, 5 mM DTT. The collected fractions were quantified by absorbance reading at 280 nm, and concentrated up to 20 mg/ml. Human Insc ∶ LGN:Gαi complexes were generated by co-infection of High5 insect cells with two baculoviruses and purified by affinity and anion exchange in the presence of Gαi obtained from bacterial sources [10] . The human Insc ∶ LGN TPR complex was expressed in High5 insect cells infected with a recombinant dicistronic baculovirus vector coding for a 6His-tagged full-length Insc (residues 1–532, Uniprot Q1MX18-2) and the fragment 15–350 of LGN (Uniprot AAB40385.1). The complex was purified on NTA beads, followed by anion exchange chromatography. For pull-down and SEC experiments, constructs encompassing the three PDZ domains of human Par3 (residues 269-685, Uniprot Q8TEW0) was cloned in pGEX-6PI, expressed in BL21 Rosetta E . Coli , and purified by affinity followed by gel filtration chromatography after GST-tag removal. Crystallization and structure determination Initial crystals of the dLGN TPR :Insc ASYM complex were obtained by sitting-drop vapor diffusion at 20 °C mixing 1 μl of the protein sample at 20 mg/ml with equal volume of a reservoir containing 20% PEG3350 and 0.2 M K-thyocianate. Optimization of the crystallization conditions resulted in plate-shaped crystals about 200 μm in size, using 1:1.5 volume ratio of protein to reservoir (13% PEG3350, 0.1 M Tris-HCl pH 7.8, 0.2 M K-thyocianate, 2.5% 1-Propanol, 2.5% Tacsimate pH 7.5) at 4 °C. For data collection, crystals were transferred to a cryo buffer (reservoir buffer supplemented with 25% glycerol), and flash-frozen in liquid nitrogen. X-ray diffraction datasets were collected to 3.4 Å and 4.0 Å resolution at I04 and I04-1 beamlines at Diamond Light Source. All data were processed with xia2 [40] . Crystals belong to the space group P2 1 2 1 2 1 . Initial phases were obtained by molecular replacement using the coordinate of dLGN TPR :Insc PEPT (PDB ID 4A1S) as search model in Phaser [41] . Automatic model building performed on the different datasets using Buccaneer [42] yielded initial models, which were employed to perform multi-crystal average density modification in Phenix [43] . The quality of the resulting electron density maps allowed building of the complete model through iterative cycles of automatic and manual model building in Phenix and Coot [44] respectively. The final model was restrained refined to R work of 20.9% and R free of 24.9%, and good stereochemistry (Table 1 ). The final model contains eight copies of dLGN TPR (residues 39–392) and Insc ASYM (residues 306 to 595) assembled in four tetramers. The structure was visualized by Pymol ( www.schrodinger.com/pymol ) and Chimera [45] . SAXS experiments SAXS data were collected using the SEC-SAXS setup at the ESRF BioSAXS beamline BM29 (Grenoble, France). 100 μl of the dLGN TPR :Insc ASYM complex at a concentration of 20 mg/ml were injected on a Superdex-200 10/30 Increase column (GE Healthcare), and 1000 individual frames of 2 s exposure were collected on the eluate using the Pilatus 1 M detector (Dectris). Individual frames were processed automatically using an EDNA based processing pipeline. Frames for further processing were chosen by selecting frames according to the match with matching radius of gyration and high similarity using CORMAP [38] . Guinier-analysis and calculation of the pair distribution function were done in Primus from the ATSAS package [46] . 20 ab initio models for both P1 and P2 symmetry were calculated using DAMMIF [47] , and then averaged, aligned and compared using DAMAVER [48] . A representative bead model was calculated using DAMMIN [49] , and aligned to the crystallographic structures using SUPCOMB and PyMol. Theoretical scattering curves of the known dLGN TPR :Insc ASYM structures were calculated and fitted to the experimental curve using WAXSiS [50] . Details of SAXS data acquisition and processing are summarized in Supplementary Table 1 . Immunoprecipitation experiments Human Insc (residues 1–532) and InscΔC (residues 1–516) were cloned into a modified version of pCDNA5 with a N-terminal HA-tag, human LGN (residues 1–677) was cloned into pCDNA5 with a C-terminal FLAG-tag, and Par3 was cloned into pEGFP_N1 (Clontech). HEK293T cells were cultured in Dulbecco’s Modified Eagle’s Medium (DMEM) supplemented with 10% of fetal bovine serum and 1% l -glutamine. Cells were transfected with the constructs indicated in the experiments, and after 48 h from transfection cells were treated with 3.3 μM of nocodazole (Sigma) for 16 h. Cell lysates prepared in JS buffer (50 mM HEPES pH 7.4, 0.15 M NaCl, 10% glycerol, 1% Triton, 1.5 mM MgCl 2 , 5 mM EGTA and protease inhibitor cocktail) were incubated with 2 mg/ml of α-FLAG M2 antibody (Sigma) or α-GFP antibody (MBL) conjugated to sepharose beads for 2 h at 4 °C. Immunopreciptated proteins were then washed four times in JS buffer, and analyzed by SDS–PAGE and immunoblotting. Human Insc ASYM (residues 1–317), GFP-Insc ASYM -ΔαB (corresponding to Insc ASYM lacking residues 62–191), GFP-LGN TPR and FLAG-LGN TPR (residues 1–350) were cloned into a pCDH vector with hygromycin resistance under a CMV promoter (CD515B System Biosciences). HEK293T cells cultured as described above were transfected with pCDH vectors expressing the different constructs as indicated in the experiments of Fig. 3f . After 48 h from transfection, cell lysates prepared in modified JS lysis buffer (50 mM HEPES pH 7.4, 0.15 M NaCl, 10% glycerol, 0,5% NP40, 1.5 mM MgCl 2 , 5 mM EGTA, 2 mM DTT and protease inhibitor cocktail) were incubated with 2 mg/ml of α-FLAG M2 antibody (Sigma) conjugated to sepharose beads for 1 h at 4 °C. Immunopreciptated proteins were then washed three times in lysis buffer, separated by SDS–PAGE, and analyzed by immunoblotting. SEC of cell lysates For experiments of Supplementary Fig. 3g , HEK293T cells cultured as described above were transfected with pCDH vectors expressing GFP-Insc ASYM and FLAG-LGN TPR constructs (generated as described in the previous paragraph) as indicated in the experiments. After 48 h from transfection, cell lysates prepared in lysis buffer (50 mM HEPES pH 7.4, 0.15 M NaCl, 10% glycerol, 0,5% NP40, 5 mM EDTA, 5 mM DTT and protease inhibitor cocktail) were filtered (0.22 μm filter) and quantified. 0.5 ml of cell lysates at a concentration of 6 μg/μl were loaded on a Superdex-200 10/30 equilibrated in 50 mM HEPES pH 7.4, 0.15 M NaCl, 10% glycerol, and 5 mM DTT. Eluted fractions were collected, separated by SDS–PAGE, and analyzed by immunoblotting. Pull-down assays Bacterially expressed GST-tagged Par3 PDZ (2 μM) was incubated with HEK293T cell lysates expressing Insc full-length or InscΔC for 2 h at 4 °C in JS buffer. After four washes in JS buffer, proteins retained on beads were resolved by SDS–PAGE, and detected by immunoblotting. Membranes were then stained with Coomassie or Ponceau to visualize the amounts of GST-fusion proteins. Mammosphere cultures Mammary tissues from p53-KO mice were processed, and primary mammospheres obtained as described [28] . Briefly, mammary tissues were mechanically dissociated and placed in a digestion medium (DMEM supplemented with 200 U/ml collagenase (Sigma) and 100 U/ml hyaluronidase (Sigma)) for 3 h at 37 °C. Cells were plated onto ultra-low attachment plates (Falcon) at a density of 50,000 viable cell/ml in a serum-free mammary epithelial basal medium (MEBM, BioWhittaker), supplemented with 5 μg/ml insulin, 0.5 μg/ml hydrocortisone, 2% B27 (Invitrogen), 20 ng/ml EGF and bFGF (BD Biosciences), and 4 μg/ml heparin (Sigma). Mammospheres were collected after 7 days and mechanically dissociated. Cells were cultured in MEBM, 0.5 mg/ml hydrocortisone, 5 μg/ml insulin, 4 μg/ml heparin (Sigma), 20 ng/ml epidermal growth factor (EGF), 20 ng/ml fibroblast growth factor (βFGF), 1% Pen/Strep, 2 mM glutamine. Mammary cells were infected with pCDH-CMV-EF1-GFP lentiviral vectors coding for Insc constructs (Insc full-length, FL; the asymmetric domain spanning residues 1–317, ASYM; and the LGN-binding peptide encompassing residues 1–58, PEPT), and selected with 2 μg/ml of puromycin in solution. To analyze MaSCs self-renewal, cells from disaggregated mammospheres grown in liquid culture were either diluted at 2000 cells/ml for serial propagation, or plated in 96 multi-well plates (1000 cells per well) in a semisolid stem cell medium supplemented with methylcellulose. Disaggregation and re-plating at the same density were repeated for three passages, at a 7-day distance. For Fig. 5e–h , cell plating in methylcellulose was performed in 10 technical replicates, which were analyzed automatically using the JMP software (SAS) to quantify mammospheres numbers, GFP intensity and diameter. For these measurements, only spheres above a 100 μm diameter size threshold were considered. To monitor Insc protein levels, cell lysates from mammosphere cultures were prepared in JS and analyzed by Western blotting using anti-Inscuteable (rabbit polyclonal, raised against fragment 1–302 of human Insc, produced in house), and anti-vinculin antibody as normalizing control (mouse monoclonal, clone hVIN-1, Sigma). Protein bands were visualized using the SuperSignal West Pico Substrate (Pierce, Rockford, IL) after incubation with an HRP-conjugated anti-mouse secondary antibody (Sigma, St. Louis, MO). For Fig. 5i , mammary cells were infected with pCDH-CMV-EF1-GFP lentiviral vectors coding for Insc constructs (Insc full-length, FL; Insc ASYM spanning residues 1–317, ASYM; and Insc ASYM -ΔαB corresponding to Insc ASYM lacking residues 62–191, ASYM-ΔαB). For experiment of Fig. 5l , mammary cells were infected with pCDH-CMV-hygro lentiviral vectors coding for mCherry or mCherry-LGN-GoLoco (residues 358–677). Cells were selected with 2 μg/mL of puromycin and 1 μg/ml hygromycin in solution. To analyze MaSCs self-renewal, cells from disaggregated mammospheres grown in liquid culture were either diluted at 2000 cell/ml for serial propagation, or plated in 24 multi-well plates (1000 cells per well) in a semisolid stem cell medium supplemented with methylcellulose. Disaggregation and re-plating at the same density were repeated for three or two passages, at a 7-day distance. Cell plating in methylcellulose was performed in four (Fig. 5i ) or three (Fig. 5l ) technical replicates. To monitor Insc protein levels, cell lysates from mammosphere cultures were prepared in JS buffer, and analyzed by western blotting using anti-Inscuteable antibody (rabbit polyclonal, raised against fragment 1–302 of human Insc, produced in house, working dilution 1:1,000), anti-mCherry (rat monoclonal, Thermo Fisher, M11217, working dilution 1:10,000)), and anti-vinculin antibody as normalizing control (mouse monoclonal, clone hVIN-1, Sigma, working dilution 1:10,000). Real-time PCR analysis Total RNA was extracted from mammary epithelial cells using Trizol (Invitrogen) and miRNeasy micro kit (QIAGEN), according to manufacturer’s instructions. Reverse-transcription was performed using the Im-Prom II Reverse Transcriptase kit for cDNA synthesis (Promega). 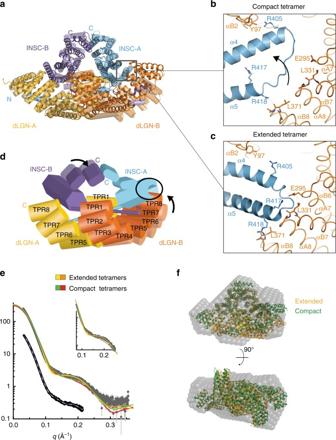Fig. 2 The dLGNTPR:InscASYMcomplex adopts two conformations.aSuperposition of the two dLGNTPR:InscASYMconformers present in the a.s.u. The most compact conformer is shown as ribbon diagram, and the most extended is depicted in transparent cylindrical helices. Subunits are colored as in Fig.1.b,cZoomed views of the interfaces between the helical bundle of Insc-Aand TPR7-8 of dLGN-Bfor the compact (top) and extended (bottom) tetramers. The rearrangement of the TPR repeats of dLGN-B in the compact conformation is accompanied by disruption of the initial turns of helix α5 of Insc-A.dGraphical summary of the conformational changes between the extended and the compact tetramers.eSAXS data for the dLGNTPR:InscASYMcomplex in comparison to the theoretical curves for the different configurations (upper part and inlay) and fits of ab initio models in P1 (gray) and P2 symmetry (blue). Idealized curves were obtained merging frames with matching radius of gyration and high similarity according to CORMAP38,39.fThe ab initio model of the dLGNTPR:InscASYMcomplex in P1 symmetry (transparent gray spheres) matches well with both the extended (orange) and compact (green) tetramers Real-time quantitative PCR (RT–qPCR) was performed with the LightCycler480 System (Roche) with the primers listed in Supplementary Table 2 . PCR efficiency of primer pairs were calculated using a standard curve to allow efficient quantification of expression and comparison of levels between different genes (Supplementary Fig. 6i ). 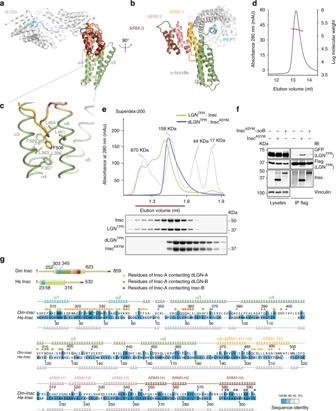Fig. 3 The topology of the asymmetric domain of Insc is evolutionary conserved.a,bCartoon model of InscASYMbound to the inner groove of dLGNTPR(in white) at two orthogonal views. After the initial InscPEPTstretch (in cyan), the Insc chain departs from the TPR α-solenoid forming a four-helix bundle (green). The C-terminal part of the last helix of the bundle kinks into two short helical fragments of the first non-canonical ARM repeat (gold), which is followed by two conventional ARM motifs adopting a triangular flat shape (pink and brown).cZoom of the hydrophobic pocket in which Phe506Inscfits.dStatic-Light-Scattering profile of the dLGNTPR:InscASYMtetramer showing an average molecular mass of about 180 kDa along the peak, as expected for a 2:2 tetramer.eSEC elution profiles ofDrosophiladLGNTPR:InscASYM(blue trace) and human LGNTPR:Insc (green trace) with associated Coomassie-stained SDS–PAGE separation of peak fractions. The elution profile of globular markers is reported in a dashed gray line. Both complexes elute in fractions consistent with the theoretical molecular mass of 2:2 tetramers.fInscASYM-ΔαB assembles with LGNTPRin a 1:1 stoichiometry. HEK293T cells were transiently transfected with plasmids containing human GFP-LGNTPRand FLAG-LGNTPR(residues 1–350) alone or in combination with human InscASYMor InscASYM-ΔαB (lacking residues 62–191). After 48 h, cells lysates were immunoprecipitated (IPs) with anti-FLAG antibodies conjugated to sepharose beads, and immunoblotted (IB) with the indicated antibodies. FLAG-LGNTPR- was able to co-immunoprecipitate with GFP-LGNTPRonly when bound to InscASYM, but not to InscASYM-ΔαB.gSequence alignment of InscASYMwith secondary structure elements based on the crystallographic structure (forDrosophila) and in silico prediction (forHomo sapiens). Residues are colored according to the degree of conservation calculated on the basis of the alignment of Supplementary Fig.4. Circles indicate residues of InscASYMin contact with the other three subunits of the tetramer Notably, mmInsc primers recognizes both mouse and human Insc, and were used for RT–qPCR of Fig. 5a , while hsInsc primers recognizes only human Insc and were used to assess the expression levels of Insc mutants in Supplementary Fig. 6 . Immunofluorescence For MaSCs doublet analyses, mammospheres were mechanically dissociated and single cells were allowed to divide once for 30 h in stem cell medium additioned with 20% methylcellulose in order to avoid aggregation. Cells were then transferred to a poly-lysine coated glass slide (Corning) and fixed with 4% paraformaldehyde (PFA) for 20 minutes at room temperature. Then, cells were blocked in donkey serum diluted 1:5 (20%) for 15 min, and incubated with anti-CD49f antibody (working dilution 1:250; clone GoH3, cat. 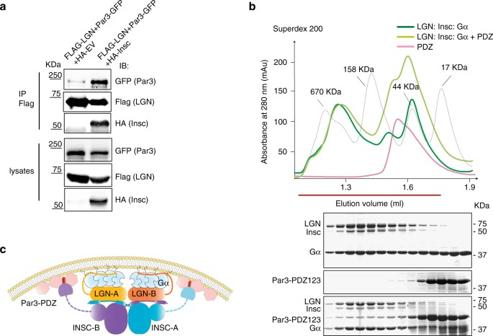Fig. 4 Conserved organizational principles of Par3:Insc:LGN:Gαi complexes.aReconstitution of human Par3:Insc:LGN interaction in cells. HEK293T cells were transfected with Par3-GFP, FLAG-LGN and HA-Insc. Cell lysates were subjected to IP with α-FLAG antibody conjugated to sepharose beads. After washes, species on beads were analyzed by SDS–PAGE and immunoblotted as indicated in the figure. HA-empty vector was included as a negative control of the IP.bSEC elution profiles and SDS–PAGE separation of Insc:LGN:Gαi complexes reconstituted from expression in insect cells (dark green trace) and Par3PDZ123purified from bacterial sources (pink trace). When the Par3PDZ123is mixed in molar excess with Insc:LGN:Gαi, it coelutes with Insc:LGN:Gαi in a stoichiometry reflecting the amount of Insc in the complex (light green trace).cSummary of the interactions in the Par3:Insc:LGN:Gαi complex supported by our study. Stable Insc:LGN tetramers form the core of apically localized Par3:Insc:LGN:Gαi complexes, in which the C-terminal portion of the two Insc chains contacts directly the PDZ domains of Par3. Binding of each LGN-GoLoco to four GαiGDPmolecules stabilizes the association of the macromolecular assemblies to the plasma membrane 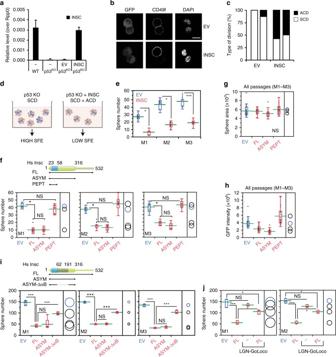Fig. 5 InscASYMinduces ACDs in p53-KO mammary stem cells.aInsc transcript levels evaluated by RT–qPCR on mammospheres from wild-type FVB mice, or p53-KO mice infected with empty lentivirus (EV) or human full-length Insc (INSC) normalized to the Rpp0 control. Bars represent mean ± s.d. of three replicates. Statistics for 1 out of 2 independent experiments.b,cImages and quantification of the division mode of mammary epithelial cells from p53-KO mice evaluated by pair-cell assay. Cell infected with empty lentivirus (EV) or virus expressing full-length Insc (INSC) were stained with CD49f and DAPI. Scale bar, 10 μm. Quantification from 2 independent experiments with n > 10 cells for all conditions in each experiment.p= 0.005 according to the paired Student’s test.dScheme of the SFE assay used to evaluate self-renewal of p53-KO MaSCs. Stem cells are in blue, progenitors in pink.eNumber of mammospheres from p53-KO mice infected with an empty lentivirus (EV) or a virus expressing Insc (INSC) counted over three serial passages and shown by box-plots with mean of 10 wells count per each passage (green line).f–hSFE assays with p53-KO mammospheres infected with empty virus (EV) or viruses expressing Insc (FL), InscASYM(aa 1–317, ASYM), or InscPEPT(aa 1–58, PEPT). For each passage, the number of spheres (f), the sphere area (g) and the GFP intensity (h) have been evaluated for 10 wells, and plotted as ine(each pair Student’st-test). Statistics for 1 out of 3 independent experiments.iSFE assays performed with p53-KO mammospheres infected with empty lentivirus (EV) or viruses expressing Insc (FL), InscASYM(ASYM), or InscASYM-ΔαB (i.e. InscASYMlacking aa 62–191). For each passage, the number of spheres has been counted for four wells, and plotted as above (each pair Student’s t-test). Statistics for one out of two independent experiments.jSFE assays performed with p53-KO mammospheres infected with empty lentivirus (EV) or viruses expressing Insc (FL), human LGN-GoLoco (aa 358–677) or both. For each passage, the number of spheres has been evaluated in three wells, and plotted as above (each pair Student’st-test). In the figure, *P< 0.01, ***P< 0.001 by Wilcoxon’s test 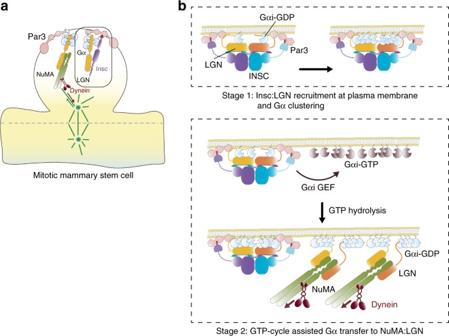Fig. 6 Model of the role of Insc:LGN complex in asymmetric divisions.aSchematic diagram depicting the organization of cortical domains and mitotic spindle motors in murine mitotic mammary stem cells.bSchematic representation of the asymmetric function of Insc:LGN tetramers supported by our study. Initally, Insc:LGN complexes are recruited at the apical membrane by direct binding of LGN to Gαi-GDP molecules, and by association of Insc with Par3. Cooperative binding to LGN-GoLoco motifs favors Gαi-GDP apical clustering. Later, a Gαi GTP-cycle, likely catalyzed by a GEF such as Ric-8A, dissociates Gαi from Insc:LGN, generating a localized pool of Gαi-GTP molecules, which upon GTP hydrolysis recruits LGN:NuMA:Dynein complexes at the apical site. According to this model, stable Insc:LGN assemblies couple asymmetric fate specification with apico-basal spindle orientation by Gαi-GDP transfer no 555734, BD Pharmigen) for 1 h at room temperature. For Supplementary Fig. 6d , cells were further stained with a monoclonal Numb antibody as described in Colaluca et al. [51] . Cells were washed with PBS, and later incubated with anti-rat cy3 antibody (working dilution 1:400; Jackson ImmunoResearch) for 30 min at room temperature. Following that, cells were washed again with PBS, and fixed with 4% PFA for 10 min at room temperature. After permeabilization with 0,1% Triton-X, cells were counterstained with DAPI (Sigma). Confocal microscopy was performed on a Leica TCS SP2 confocal microscope. A 63 × oil-immersion objective lens (HCX Plan-Apochromat 63× NA 1.4 Lbd Bl; Leica) was used for analysis. Data availability Data are available on request from the authors. The coordinates and structure factors of the structure are available from the Protein Data Bank under the accession number 5A7D.